Doped organic transistors operating in the inversion and depletion regime The inversion field-effect transistor is the basic device of modern microelectronics and is nowadays used more than a billion times on every state-of-the-art computer chip. In the future, this rigid technology will be complemented by flexible electronics produced at extremely low cost. Organic field-effect transistors have the potential to be the basic device for flexible electronics, but still need much improvement. In particular, despite more than 20 years of research, organic inversion mode transistors have not been reported so far. Here we discuss the first realization of organic inversion transistors and the optimization of organic depletion transistors by our organic doping technology. We show that the transistor parameters—in particular, the threshold voltage and the ON/OFF ratio—can be controlled by the doping concentration and the thickness of the transistor channel. Injection of minority carriers into the doped transistor channel is achieved by doped contacts, which allows forming an inversion layer. Controlled doping of semiconductors leads to highly reproducible transistors with precisely tunable device characteristics [1] , which is witnessed by the success of inorganic metal-oxide-semiconductor field-effect transistors. However, most surprisingly, organic field-effect transistors (OFETs) almost exclusively use electrically undoped semiconductors and OFETs with doped channels are rarely reported. Doping has only been used to realize depletion type OFETs [2] , [3] , [4] , [5] , [6] , [7] , [8] , [9] , [10] . In these devices, doping either results in a low ON/OFF ratio for higher dopant concentrations, or the effect of doping on the transistor behaviour, for example, on the threshold voltage, is limited when lower concentrations are chosen [3] , [5] . In contrast to depletion type transistors organic inversion transistors, that is, transistors in which, for example, a p-inversion layer is created in an n-doped channel layer, have not been realized so far. The main challenge of reaching the inversion regime is the generation of minority charge carriers at the interface to the gate insulator. Scheinert et al. [11] have argued that the inversion regime in organic metal-insulator-semiconductor (MIS) capacitances cannot be reached due to the large time constant of minority charge carrier generation. Scheinert et al. [11] and Lindner et al. [12] also proposed theoretically that minority charge carriers could be injected from the source of the OFET into the channel, if injection is efficient. However, Brondijk et al. [13] recently showed that injection of minority charge carriers in P3HT-based transistors is too inefficient in order to generate an inversion channel. Here, we report both inversion and depletion OFETs. Depletion OFETs with high ON/OFF ratio are realized by keeping the doped layer as thin as possible, that is, a few nanometres only, which allows for a full depletion of the doped region by the applied gate voltage. Organic inversion transistors are facilitated by additionally doping of the source and drain contact, which leads to efficient injection of charge carriers and allows for the creation of an inversion layer. We show that doping leads to a precise control of the threshold voltage of OFETs. Controlling and stabilizing the threshold voltage in OFETs is essential in the design and production of larger integrated circuits. In particular, small and symmetric threshold voltages for p- and n-type transistors are needed for low-power complementary circuits. Doping of pentacene by the p-dopant F 6 TCNNQ and the n-dopant W 2 (hpp) 4 Owing to its high hole mobility, pentacene is chosen as organic matrix material. F 6 TCNNQ is used as p-dopant, which shows a similar doping strength as the commonly used dopant F 4 TCNQ. F 6 TCNNQ, however, has a higher molecular weight, which allows a more precise control during evaporation and makes molecular diffusion of the dopant less probable [14] . As n-dopant, W 2 (hpp) 4 is used, which is also well known to significantly increase the conductivity of the fullerene C 60 (ref. 15 ). To prove that pentacene is p- as well as n-dopable and to distinguish between trap filling by doping and real doping, that is, generation of free charges, we study the shift of the Fermi level upon doping by ultraviolet photoelectron spectroscopy (UPS). 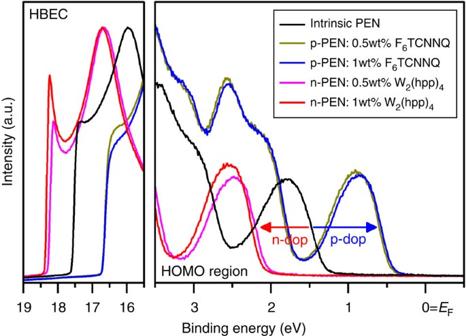Figure 1: Doping of pentacene studied by ultraviolet photoelectron spectroscopy. Pentacene (PEN) is doped by F6TCNNQ (p-doping) and W2(hpp)4(n-doping) (HBEC: high binding energy cutoff). The shift of the HOMO of pentacene relative to the Fermi level (at 0 eV) is strong already at a low doping concentration of 0.5 wt%. For p-doping, the HOMO shifts towards the Fermi level and for n-doping away from the Fermi level. Figure 1 shows the UPS spectrum for 45 nm of pentacene, which is either intrinsic, doped by 0.5 wt% or 1 wt% of the p-dopant F 6 TCNNQ, or doped by 0.5 wt% or 1 wt% of the n-dopant W 2 (hpp) 4 . To avoid any reactions at the substrate surface (silver) and to make the growth of pentacene more reproducible, a 4 nm interlayer of MeO-TPD is included between the silver substrate and pentacene. Figure 1: Doping of pentacene studied by ultraviolet photoelectron spectroscopy. Pentacene (PEN) is doped by F 6 TCNNQ (p-doping) and W 2 (hpp) 4 (n-doping) (HBEC: high binding energy cutoff). The shift of the HOMO of pentacene relative to the Fermi level (at 0 eV) is strong already at a low doping concentration of 0.5 wt%. For p-doping, the HOMO shifts towards the Fermi level and for n-doping away from the Fermi level. Full size image Figure 1 shows that the highest occupied molecular orbital (HOMO) states shift strongly towards the Fermi level (at 0 eV) for p-doping and away from the Fermi level for n-doping. The work function of the films and the difference between the Fermi level and the HOMO of pentacene η for the different doping concentrations are summarized in Table 1 . For the intrinsic material, the Fermi level is close to the midgap position ( η =1.31 eV, ionization potential=4.94 eV). Already at a dopant concentration of 0.5 wt% doping leads to a strong Fermi level shift towards the HOMO for p-doping ( η =0.46 eV) and away from the HOMO for n-doping ( η =2.05 eV), whereas the ionization potential of pentacene remains almost unchanged. Further increase of the dopant concentration leads only to a weak additional shift of the Fermi level ( η =0.43 eV for 1 wt% of p-doping and η =2.12 eV for 1 wt% of n-doping). These observations are in qualitative agreement with doping of the organic light-emitting diode (OLED) hole transport material MeO-TPD by F 4 TCNQ [16] , F 6 TCNNQ or C 60 F 36 (ref. 17 ). Most importantly, the strong shift of the Fermi level towards the transport states indicates that free charges are generated. If doping would only fill traps the Fermi level would be pinned at the trap level, an effect observed, for example, at low concentrations in MeO-TPD [17] . Table 1 Doping of pentacene studied by UPS. Full size table Depletion transistors To realize depletion transistors, source and drain contact as well as the channel are p-doped. To keep the ON/OFF ratio of the intrinsic transistor, only a thin layer (6 nm) at the interface between gate oxide and pentacene layer is doped. The general set-up for the transistors is sketched in Fig. 2 . They consist of aluminium gate electrodes, 120 nm of Al 2 O 3 dielectric layer deposited by atomic layer deposition (ALD), a thin p-doped layer of pentacene (6 nm, intrinsic, 0.5, 1 and 2 wt% F 6 TCNNQ), and 40 nm of intrinsic pentacene. The intrinsic layer ensures a fully closed pentacene layer, even if the thickness of the doped pentacene layer is decreased in later experiments. The source and drain contacts are defined by shadow masks and consist of 50 nm of p-doped pentacene (F 6 TCNNQ, 4 wt%) to ensure efficient injection and 50 nm of aluminium. Figure 3a shows the transfer characteristics of these transistors with varying doping concentrations in the channel. 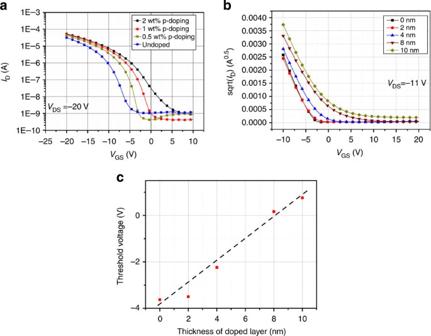Figure 3: Organic depletion transistors. (a) Transfer characteristics of depletion transistors with a 6 nm p-doped channel at varying concentrations (0, 0.5, 1 and 2 wt% F6TCNNQ,VDS=−20 V). The transfer characteristic is consistently shifted to the right and the threshold voltage decreases. Inb, the thickness of the doped channel at a constant doping concentration (2 wt%) is varied. Thicker layers lead to a stronger shift of the threshold voltages plotted in partc. The thickness dependence of the threshold voltage shift proves that the effect is not due to trap filling at the oxide/organic interface. All devices are processed in a single deposition run, for example, on the same substrate and at identical deposition conditions, which minimizes experimental uncertainties in the comparison of the devices. As can be seen in Fig. 3a , the transfer characteristic shifts consistently towards more positive voltages upon increasing p-doping concentrations and the threshold voltage decreases. Most importantly, all doped samples show the same ON/OFF ratio, that is, the doped layer can be fully depleted. The 0.5 and 1 wt% sample even show a slightly increased ON/OFF ratio, which, however, is most probably due to sample to sample variations. Only at the highest doping concentration (2 wt%), the performance and in particular the subthreshold swing of the transistor degrades. 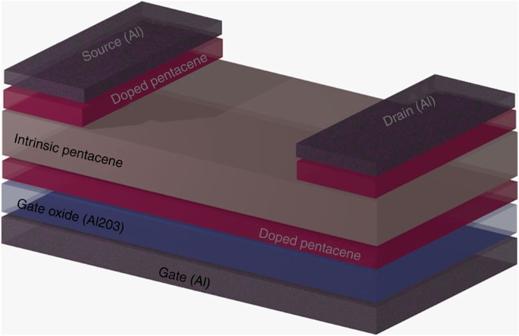The devices show moderate hole mobilities in the order of 0.1 cm 2 (Vs) −1 , which can be explained by the high-k dielectric, which is known to reduce the mobility in OFETs [18] , and by the deposition at room temperature. Figure 2: Doped OFETs. Set-up of the transistors consisting of Al2O3as gate oxide, a thin doped layer of pentacene as transistor channel, an intrinsic pentacene layer and doped source and drain contacts. Figure 2: Doped OFETs. Set-up of the transistors consisting of Al 2 O 3 as gate oxide, a thin doped layer of pentacene as transistor channel, an intrinsic pentacene layer and doped source and drain contacts. Full size image Figure 3: Organic depletion transistors. ( a ) Transfer characteristics of depletion transistors with a 6 nm p-doped channel at varying concentrations (0, 0.5, 1 and 2 wt% F 6 TCNNQ, V DS =−20 V). The transfer characteristic is consistently shifted to the right and the threshold voltage decreases. In b , the thickness of the doped channel at a constant doping concentration (2 wt%) is varied. Thicker layers lead to a stronger shift of the threshold voltages plotted in part c . The thickness dependence of the threshold voltage shift proves that the effect is not due to trap filling at the oxide/organic interface. Full size image These results show that the threshold voltage can be controlled by doping. The shift can be caused by two mechanisms: First, doping increases the density of free holes in the channel region. To reach the same density of free charges in the undoped transistors, an additional voltage of has to be applied to the gate ( N A , doping concentration; d dop , thickness of doped film; C ox , capacitance of gate oxide; e , elementary charge). Thus, one can define the threshold voltage of the doped transistor as ( V FB , flatband voltage of transistors) Alternatively, the shift of the threshold voltage can also be explained by a filling of traps as proposed by Olthof et al. [10] They showed that doping at ultralow concentrations fill traps in the n-type semiconductor C 60 reducing the threshold voltage in these devices while keeping the ON/OFF ratio of the transistor [10] . Similarly, Naab et al. [19] showed that filling of traps in TIPS-pentacene by an n-dopant facilitates a high electron mobility in TIPS-pentacene (6,13-Bis(triisopropylsilylethynyl)pentacene). However, the UPS results of p- and n-doped pentacene films discussed above show that doping is effective. The Fermi Level shifts strongly towards the transport states, even at relatively low concentrations of 0.5–2 wt%, proving that free charge carriers are generated in the bulk of pentacene. Nevertheless, the shift of the flat band voltage could also be caused by a filling of traps at the interface between gate oxide and pentacene. To figure out if trap filling at the organic/gate oxide interface has a significant effect on the threshold voltage, we vary the thickness of the doped layer from 2 to 10 nm. Intentionally, we keep the doping concentration at a high level of 2 wt% to enhance the effect, which however leads to a slight deterioration of the performance of individual transistors, in particular to a reduction in mobility of pentacene to ~0.06 cm 2 (Vs) −1 . This effect can be explained by a structural phase transition of the pentacene film from crystalline to amorphous [20] . Figure 3b shows the result of this experiment. As expected, the undoped reference device (black line) exhibits typical p-type transistor behaviour with a threshold voltage of approximately −3.6 V. Higher positive voltages have to be applied to the gate to fully deplete the transistor for increasing thickness of the doped channel layer. For a 10 nm doped layer, a full depletion cannot be reached any more, but for thinner layers the same off-current level as well as the same ON/OFF ratio of almost five orders of magnitude are reached. This conclusion is in accordance with previous studies of pentacene-based OFETs, where it was shown that carrier transport for undoped pentacene happens in the few first pentacene/oxide interfacial layers [21] . More importantly, the threshold voltage shifts with increasing thickness of the doped layer. This shift is proportional to the number of free charges in the doped layer ( cf . equation (1)), which is shown in Fig. 3c plotting the threshold voltage as determined by a linear fit of Fig. 3b in the range of −10 to −5 V versus the thickness of the doped layer. The threshold voltage shifts linearly from −3.6 V for the undoped transistor to 0.8 V for the 10-nm thick doped layer. Assuming a dielectric constant of the Al 2 O 3 layer of 7.8, a density of free charge carriers in the doped layer of ~2.6 × 10 18 cm −3 is determined by equation (1). This carrier density corresponds to a doping efficiency (density of free holes divided by density of dopants) of 5.9%, which is in the same order of magnitude as the doping efficiency observed in other material systems [16] . In summary, the linear shift of the threshold voltage with the thickness of the doped layer clearly shows that the shift of threshold voltage is not due to filling of traps at the organic/gate oxide interface, but due to a real doping of free charges into the channel. Inversion transistors In contrast to organic depletion transistors, organic inversion transistors have not yet been reported in the literature. The lack of inversion has been explained by inefficient injection of minority charge carriers into the inversion channel [13] . However, in our design we have the possibility to selectively dope the source drain region and to facilitate efficient injection, for example, of holes into a p-type inversion channel formed in an n-doped channel region. The formation of the inversion channel is studied by capacitance–voltage (CV) measurements as shown in Fig. 4a . The samples consist of aluminium back electrodes, 120 nm of Al 2 O 3 , a thin n-doped layer of pentacene (6 nm, intrinsic, 0.5, 1 and 2 wt% W 2 (hpp) 4 ), 40 nm of intrinsic pentacene, 200 nm of p-doped pentacene (F 6 TCNNQ, 4 wt%) to ensure efficient hole injection or 200 nm of n-doped pentacene (W 2 (hpp) 4, 2 wt%) to allow for electron injection, and 50 nm of aluminium. The voltage is applied to the injecting contact and the back contact is kept at ground potential. All samples have been processed in a single deposition run to ensure highest reproducibility. Furthermore, care has been taken to characterize the different samples at identical conditions, that is, at the same maximum voltage, to make sure the shift of the characteristic is not due to different trapping/detrapping of doped electrons at the oxide/organic interface [22] . 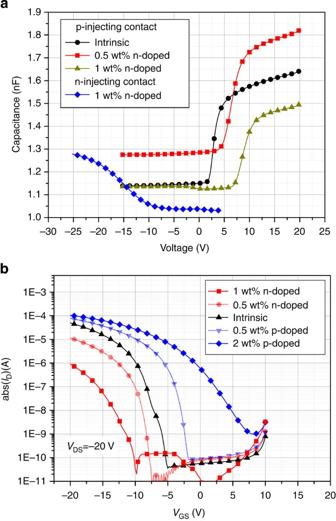Figure 4: Organic inversion transistors. (a) CV characteristic of capacitors consisting of 120 nm Al2O3, a 6 nm n-doped pentacene film, an intrinsic pentacene layer and a hole (p-doped) injecting or electron (n-doped) injecting contact. Partbshows the transfer characteristic of transistors using the same gate stack and hole injecting contacts. For comparison, p-doped depletion transistors are shown as well. Figure 4: Organic inversion transistors. ( a ) CV characteristic of capacitors consisting of 120 nm Al 2 O 3 , a 6 nm n-doped pentacene film, an intrinsic pentacene layer and a hole (p-doped) injecting or electron (n-doped) injecting contact. Part b shows the transfer characteristic of transistors using the same gate stack and hole injecting contacts. For comparison, p-doped depletion transistors are shown as well. Full size image The intrinsic sample shows a depletion region at negative voltages and accumulation at positive voltages. N-doping the channel but keeping the hole injecting contact leads to a shift of the characteristic to more positive voltages. The shift of the characteristic is increased for increasing doping concentration. Changing from p-injecting contacts to n-injecting contacts allows observing accumulation of electrons as well at negative voltages (blue line in Fig. 4a ). Transistors built using the same stack show the same trends ( cf . Fig. 4b ). All samples have p-injecting contacts. The inversion transistors have a 6-nm thick n-doped channel. P-doped depletion transistors processed in the same run are shown for comparison as well. As seen in Fig. 4b , the n-doped transistors clearly show a p-type characteristic, that is, the transistor turns on at negative voltages. In accordance with the CV characterization, the threshold voltage increases for increasing n-doping concentration. This shift of the CV characteristic and the shift of the threshold voltage can be explained by an inversion of the n-doped layer at the oxide/pentacene interface. An increased potential has to be applied to the sample to first deplete the n-doped layer and to subsequently form an inversion layer of holes at even higher voltages. By increasing the density of n-dopants into the channel, more voltage has to be applied to the gate to reach inversion and the threshold voltage increases. Our results show that organic depletion and inversion transistors can be realized by doping a very thin layer of the organic semiconductor pentacene at the interface to the gate oxide. Doping leads to highly reproducible and tunable device characteristic. In particular, the threshold voltage of the transistors can be actively controlled by the thickness of the doped layer or the doping concentration while keeping other performance parameter such as the ON/OFF ratio, the sub-threshold swing and the mobility of pentacene constant. Owing to the precisely tunable device characteristics, we anticipate that doping in organic transistors will, similar to doping in inorganic transistors, become a key technology easing the design of larger integrated organic circuits. Device fabrication All samples are prepared by thermal evaporation in a single-chamber UHV tool (Kurt J. Lesker Company) at a base pressure of 10 −7 mbar. The deposition system is equipped with a wedging tool, which allows depositing several samples with systematic variations on the same substrate in a single deposition run ensuring best comparability of the samples. Four different processing runs are processed to reproduce the results, each consisting of 12 different transistors with slightly varied processing parameters. Despite some substrate to substrate variations, all runs show the same trends. The transistors show a small hysteresis between forward and backward sweep of 1–2 V only. The samples consist of 60 nm Al as gate, 120 nm Al 2 O 3 as gate oxide, a thin layer of pentacene (0–10 nm, Sensient, Wolfen, Germany, density 1.32 g cm −3 , M W =278.35 g mol −1 ) doped either with the p-dopant F 6 TCNNQ (2,2′-(perfluoronaphthalene-2,6-diylidene)dimalononitrile) or the n-dopant W 2 (hpp) 4 (tetrakis(1,3,4,6,7,8-hexahydro-2H-pyrimido[1,2-a]pyrimidinato)ditungsten (II), both Novaled AG). On top of the doped layer, 40 nm of intrinsic pentacene is deposited. The source and drain contact consist of a doped pentacene layer (50 nm ( Fig. 3 ) or 200 nm ( Fig. 4 ) doped with F 6 TCNNQ at 4 wt%) and 50 nm Al. The bulky molecular dopants F 6 TCNNQ and W 2 (hpp) 4 are used to avoid diffusion of dopants and instable doping profiles. In pin junctions, we were able to show by impedance spectroscopy that equivalent dopants show negligible diffusion and form sharp doping profiles [23] . Similarly, He et al. [24] could show that proprietary n-dopants of Novaled AG do not show strong diffusion, even under applied electrical field. Nevertheless, owing to the rough morphology of pentacene, we cannot exclude that the interface between the doped and intrinsic layer underneath the source and drain contacts is not as flat as shown in the sketch of the device in Fig. 2 . The transistors are structured by shadow masks with a channel length of 300 μm and a channel width of 20 mm. Glass is used as substrate. Before transferring the samples to air, the samples are encapsulated under nitrogen atmosphere. The Al 2 O 3 layers are deposited in a cross-flow ALD reactor, which is part of an FHR Anlagenbau ALD 300 cluster system. Both, deposition process and film properties were optimized using in situ quartz crystal microbalance and in situ X-ray photoelectron spectroscopy. The deposition of aluminium oxide is carried out with the precursors trimethylaluminum (Al(CH 3 ) 3 ) and ozone. The two pulses (2 s Al(CH 3 ) 3 and 4 s ozone) are separated by Ar purge pulses (2 s). The precursors are pulsed into a constant flow of 400 sccm Ar. The oxide layers are grown at 200 °C, yielding a growth rate of 0.11 nm per cycle. The Al 2 O 3 is deposited onto the glass substrates covered by the gate structures (aluminium). Device characterization The capacitance versus voltage characteristic shown in Fig. 4a is done using an HP 4284 A Precision LCR meter. The CV sweep has been measured at a modulation amplitude of 20 mHz and at a frequency of 100 kHz. Care has been taken to measure the capacitances (and transistors as well) at identical conditions, in particular at identical voltages. Characterization of the electrical characteristic of the transistors is done using the Semiconductor Parameter Analyzer Keithley 4200-SCS. All electrical measurements are performed at room temperature. All devices are stable under repeated cycling. To ensure a high comparability, all transfer characteristics of a series are measured at constant V DS . UPS on doped layers The UPS samples are prepared by thermal evaporation under high vacuum conditions (base pressure 10 −8 mbar) at room temperature in a multi-chamber tool. The doped layers are processed by co-evaporation of the matrix and dopant materials controlled by two independent quartz crystal microbalances. Pentacene was sublimed threefold and MeO-TPD [N,N,N′,N′-Tetrakis(4-methoxyphenyl)-benzidine] (Sensient) fourfold. The dopant materials F 6 TCNNQ and W 2 (hpp) 4 are purchased from Novaled AG. As substrate a sputter-cleaned silver foil (99.995%, MaTecK) is used. The UPS measurements are performed with a Phoibos 100 system (Specs) under ultra high vacuum conditions at a base pressure of 10 −10 mbar. Sample transfer without breaking the vacuum conditions is ensured by a direct connection of the UPS chamber to the evaporation tool. The energy resolution for UPS (HeI, 21.22 eV) is 130 meV and the experimental error (reproducibility) is estimated to 50 meV. During the UPS measurement the sample is set to an acceleration potential of −8 V. For each spectrum, the emission features due to secondary line excitations of the HeI discharge lamp are subtracted [17] . For each sample the work function, defined as W f =21.22 eV – high binding energy cutoff (HBEC) as well as the HOMO – onset relatively to the Fermi level of the substrate are determined from the UPS spectrum. The measurements are kept as short as possible to avoid ultraviolet degradation of the organic materials. How to cite this article: Lüssem, B. et al. Doped organic transistors operating in the inversion and depletion regime. Nat. Commun. 4:2775 doi: 10.1038/ncomms3775 (2013).